Tailoring the topology of an artificial magnetic skyrmion Despite theoretical predictions, it remains an experimental challenge to realize an artificial magnetic skyrmion whose topology can be well controlled and tailored so that its topological effect can be revealed explicitly in a deformation of the spin textures. Here we report epitaxial magnetic thin films in which an artificial skyrmion is created by embedding a magnetic vortex into an out-of-plane aligned spin environment. By changing the relative orientation between the central vortex core polarity and the surrounding out-of-plane spins, we are able to control and tailor the system between two skyrmion topological states. An in-plane magnetic field is used to annihilate the skyrmion core by converting the central vortex state into a single domain state. Our result shows distinct annihilation behaviour of the skyrmion core for the two different skyrmion states, suggesting a topological effect of the magnetic skyrmions in the core annihilation process. A skyrmion is a topological twist of a continuous field that was first proposed by Skyrme [1] , [2] to describe discrete nucleons. In condensed-matter physics, skyrmions emerge as topological invariant spin textures in a two-dimensional Heisenberg spin lattice [3] . Evidence of skyrmions in condensed matter physics appeared after the discovery of the Quantum Hall Effect in which the lowest energy charged excitations can be mapped onto two-dimensional magnetic skyrmion states [4] , [5] . Although great effort has been made thereafter to understand the skyrmion effect in condensed matter physics, it was only recently considered that magnetic skyrmions may exist in real materials. The breakthrough occurred when it was proposed [6] that the Dzyaloshinsky–Moriya (DM) interaction [7] could compete with the Heisenberg collinear interaction to stabilize a skyrmion lattice in magnetic materials lacking inversion symmetry. Soon after this theoretical prediction, magnetic skyrmions were identified in a narrow part of a phase diagram by neutron diffraction [8] and later further confirmed by direct imaging in real space [9] , [10] . These newly discovered skyrmion materials [11] exhibit many fascinating phenomena such as the topological electric [12] , [13] , [14] and spin [15] , [16] Hall effects, specific heat anomaly [17] , skyrmion motions [18] , [19] and excitations [20] , [21] , dynamics [22] , [23] , switching [22] and the topological knots of spin textures [24] , [25] and so on. It is well recognized that these newly discovered skyrmion materials have opened a new field for the study of topological effect in fundamental physics [26] , [27] . Despite this rapid progress, however, constraints on the existence of the skyrmions (for example, the limited range of magnetic field, temperature, length scale and so on) have been demanding an experimental realization of robust skyrmions whose topology can be well controlled and tailored in a wider range of parameter space so that topological effects can be directly revealed in the deformation of the spin textures. As outlined in ref. 11 , there exist four general approaches to realize skyrmions: magnetic dipolar interaction, the DM interaction, frustrated exchange interactions or four-spin exchange interactions. In particular, the method based on the dipolar interaction could lead to the formation of skyrmions in centrosymmetric magnetic thin films [28] , [29] . For example, it is recently shown that the so-called magnetic bubbles [30] in M-type ferrite thin films are actually magnetic skyrmions with rich topological structures [29] . Recognizing that an out-of-plane magnetic bubble in a perpendicularly magnetized thin film can be deformed smoothly into a magnetic vortex (including the out-of-plane vortex core) surrounded by an out-of-plane magnetized background, it is easy to understand the recent theoretical proposal that embedding a magnetic vortex state [31] into an out-of-plane magnetized environment could lead to the formation of an artificial skyrmion [32] . The challenging questions are: is it possible to realize such an artificial skyrmion in experiment; how to control and tailor its topologies; and what kind of topological effect can be retrieved from this engineered state? In this study, we report our experimental result on the realization of this type of artificial skyrmion by growing an epitaxial Co vortex disk on top of an out-of-plane magnetized Ni film. We show that we can control the skyrmion topological index of this system and subsequently reveal the topological effect in a skyrmion core annihilation process. Experimental design We fabricated 30-nm-thick Co circular disks (radius=1 μm) on top of a 30 monolayer (Ml) thick Ni film, which was grown epitaxially on a Cu(001) substrate. It is well known [33] that epitaxial Ni/Cu(001) has an out-of-plane magnetization above ~7 Ml Ni thickness, Co/Cu(001) film has an in-plane magnetization and Co/Ni(30 Ml)/Cu(001) magnetization undergoes a spin re-orientation transition from out-of-plane to in-plane direction as the Co thickness increases above ~1 nm. Magneto-Optic Kerr Effect (MOKE) measurement on Co/Ni(30 Ml)/Cu(001) continuous film shows that the Co/Ni(30 Ml) film exhibits only the polar hysteresis loop (magnetic field applied in the out-of-plane direction) with a full remanence for Co thickness <1 nm, and only the longitudinal hysteresis loop (magnetic field applied parallel to the film plane) with a full remanence for Co thickness thicker than 1 nm, confirming that the Co/Ni(30 Ml)/Cu(001) magnetization changes from out-of-plane to in-plane direction as the Co thickness increases above ~1 nm ( Fig. 1 ). 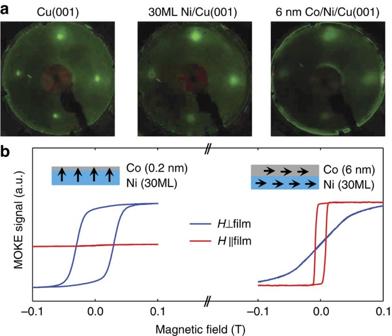Figure 1: Low-energy electron diffraction (LEED) patterns and hysteresis loops of Co/Ni(30 Ml)/Cu(001). (a) LEED patterns confirm the formation of epitaxial single crystalline films. (b) MOKE hysteresis loops show that the Co/Ni(30 Ml)/Cu(001) film has an out-of-plane magnetization for Co film thinner than 1 nm and an in-plane magnetization for Co film thicker than 1 nm. Figure 1: Low-energy electron diffraction (LEED) patterns and hysteresis loops of Co/Ni(30 Ml)/Cu(001). ( a ) LEED patterns confirm the formation of epitaxial single crystalline films. ( b ) MOKE hysteresis loops show that the Co/Ni(30 Ml)/Cu(001) film has an out-of-plane magnetization for Co film thinner than 1 nm and an in-plane magnetization for Co film thicker than 1 nm. Full size image Therefore, our Co(disk)/Ni(30 Ml)/Cu(001) sample should consist of two distinct regions in terms of magnetization direction: (1) the Co/Ni disk has an in-plane magnetization and (2) the Ni surrounding the disk has an out-of-plane magnetization. Element-specific X-ray magnetic circular dichroism (XMCD) measurements ( Fig. 2 ) confirm this spin configuration that the Co exhibits an in-plane magnetic hysteresis loop with a full remanence and the surrounding Ni exhibits an out-of-plane magnetic hysteresis loop with a full remanence (the Ni XMCD measures only the Ni region surrounding the Co disks because of the surface sensitivity of the XMCD measurement). 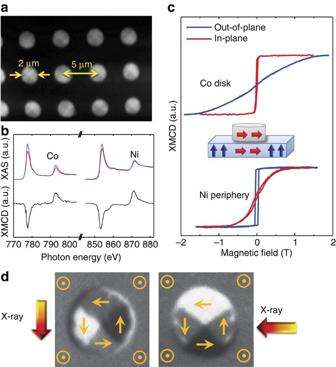Figure 2: Element-specific magnetic measurement of the Co disk and the surrounding Ni. (a) PEEM image of the Co(disk)/Ni(30 Ml)/Cu(001) sample fabricated using shadow mask. (b) X-ray absorption spectra (XAS) of Co and Ni at 2p levels for left circular polarized X-ray. The difference of the XAS for magnetization parallel (red colour) and antiparallel (blue colour) to the X-ray beam represents the element-specific XMCD signal. (c) Element-specific hysteresis loops shows that the Co disk (together with the Ni below the disk) has an in-plane magnetization and the Ni surrounding the disk has an out-of-plane magnetization. (d) Co PEEM images with different X-ray incident directions show that the Co disk in Co(disk)/Ni(30 Ml)/Cu(100) forms a magnetic vortex state. The central vortex plus the surrounding out-of-plane Ni spins correspond to a magnetic skyrmion32. Figure 2: Element-specific magnetic measurement of the Co disk and the surrounding Ni. ( a ) PEEM image of the Co(disk)/Ni(30 Ml)/Cu(001) sample fabricated using shadow mask. ( b ) X-ray absorption spectra (XAS) of Co and Ni at 2p levels for left circular polarized X-ray. The difference of the XAS for magnetization parallel (red colour) and antiparallel (blue colour) to the X-ray beam represents the element-specific XMCD signal. ( c ) Element-specific hysteresis loops shows that the Co disk (together with the Ni below the disk) has an in-plane magnetization and the Ni surrounding the disk has an out-of-plane magnetization. ( d ) Co PEEM images with different X-ray incident directions show that the Co disk in Co(disk)/Ni(30 Ml)/Cu(100) forms a magnetic vortex state. The central vortex plus the surrounding out-of-plane Ni spins correspond to a magnetic skyrmion [32] . Full size image Static measurements of skyrmion The Co magnetic domain image from photoemission electron microscopy (PEEM) measurement clearly shows the formation of magnetic vortex state (spins curling around the centre of the vortex). The vortex contrast changes accordingly after changing the in-plane projection of the X-ray beam by 90 o ( Fig. 2d ), confirming that the vortex state is an in-plane curling of the spin texture (the observation of the out-of-plane vortex core is beyond the PEEM spatial resolution). It should be mentioned that the 30-nm Co disk prevents a direct imaging of the Ni domain beneath the Co disk because of the PEEM surface sensitivity. However, the MOKE result ( Fig. 1 ) and previous works [34] , [35] in the literature show that the strong Co/Ni interfacial coupling makes the Co/Ni bilayer behave as a single ferromagnetic layer with the same domain pattern. This assertion is further confirmed by our micromagnetic simulations (see below). Thus, we conclude that the Ni region beneath the Co disk follows the same Co vortex structure. This creates a magnetic system in which the Co disk (together with the Ni below the disk) forms an in-plane magnetic vortex with the Ni spins surrounding the disk having an out-of-plane magnetization. Note that an isolated magnetic vortex is half of a skyrmion [36] and that a vortex connected to an out-of-plane spin environment is a full skyrmion; our system of the central vortex connected to the out-of-plane surrounding Ni spins thus corresponds exactly to the skyrmion spin texture proposed in ref. 32 . The topology of a skyrmion is characterized by an integer index (the so-called skyrmion number) [11] where is the normalized magnetization field ( ). The beauty of the skyrmion topology is that the skyrmion number is topologically invariant against a smooth deformation of the spin texture. In particular, the two skyrmion textures for a central vortex surrounded by out-of-plane spins have indices of N =0 and N =1, which are determined only by the central vortex core polarity relative to the surrounding out-of-plane spins ( N =0 for parallel alignment and N =1 for antiparallel alignment) regardless of the spin texture details [11] , [37] . In our experiment, we realize the N =0 state by first applying a H =20,000 Oe magnetic field in the out-of-plane direction and then turning off the field. As both the Ni film and the Co disk have an out-of-plane saturation field <20,000 Oe ( Fig. 2 ), the central vortex core polarity after turning off the magnetic field will be parallel to the surrounding Ni spins to form the N =0 state ( Fig. 3b ). To prepare the N =1 skyrmion state, we apply an 800-Oe magnetic field to the N =0 state in the opposite direction of the original 20,000 Oe direction (for example, opposite to the core polarity direction) and then turn off the field. As the magnetic coercivity of the surrounding Ni is 500 Oe and the core polarity reversal field for a permalloy disk is >3,000 Oe [38] (our simulation result shows that the vortex core switching field for our Co/Ni disk should be ~6,000 Oe), the 800-Oe field will only reverse the surrounding Ni spin direction without reversing the central vortex core polarity. Therefore, the ending state has opposite orientation between the central vortex core polarity and the surrounding Ni spins, that is, the N =1 skyrmion state ( Fig. 3b ). We performed micromagnetic simulations using the parameters of our experimental system. 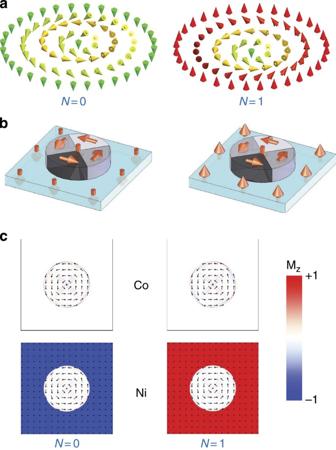Figure 3: A magnetic skyrmion consists of a central in-plane vortex and the surrounding out-of-plane spins. (a)N=0 state andN=1 skyrmion state are characterized by a parallel and antiparallel alignment of the central vortex core polarity relative to the surrounding out-of-plane spins, respectively. (b)N=0 state andN=1 skyrmion state in Co(disk)/Ni(30 Ml)/Cu(100) can be prepared by switching the surrounding Ni spin direction without switching the central vortex core polarity using an 800-Oe out-of-plane magnetic field. (c) Micromagnetic simulation confirms the formation ofN=0 state andN=1 skyrmion state by switching the surrounding Ni spin direction without changing the core polarity (blue dot at the centre). Figure 3c shows the simulation result of the Co and Ni remanent domains after applying a 20,000-Oe out-of-plane magnetic field in the − z direction and subsequently a 1,000-Oe out-of-plane magnetic field in the + z direction. The simulation result clearly shows the formation of skyrmions in the Ni film. In fact, numerical calculation of the skyrmion number using equation (1) from the Ni spin texture in Fig. 3c yields N =0.0001 for skyrmion core parallel to the surrounding Ni spins and N =0.9965 for skyrmion core antiparallel to the surrounding Ni spins. Figure 3: A magnetic skyrmion consists of a central in-plane vortex and the surrounding out-of-plane spins. ( a ) N =0 state and N =1 skyrmion state are characterized by a parallel and antiparallel alignment of the central vortex core polarity relative to the surrounding out-of-plane spins, respectively. ( b ) N =0 state and N =1 skyrmion state in Co(disk)/Ni(30 Ml)/Cu(100) can be prepared by switching the surrounding Ni spin direction without switching the central vortex core polarity using an 800-Oe out-of-plane magnetic field. ( c ) Micromagnetic simulation confirms the formation of N =0 state and N =1 skyrmion state by switching the surrounding Ni spin direction without changing the core polarity (blue dot at the centre). Full size image Annihilation of skyrmion To reveal the topological effect of the skyrmion, we studied the skyrmion core annihilation by applying an in-plane magnetic field of various strengths. Within an in-plane magnetic field, the skyrmion core moves sideways to expand the domain parallel to the field [39] . If the in-plane field is not strong enough to push the core out of the disk (for example, annihilate the skyrmion core), the skyrmion core will move back to the disk central region after turning off the field. On the other hand, if the in-plane field reaches a critical field to annihilate the skyrmion core by pushing it out of the disk region, the disk region will be converted from a vortex state to a single domain state. As the Co dots have the radius of 1 μm and thickness of 30 nm, which lead to a bistable phase of Co domain within the disk region (vortex state and single domain state are both stable under zero magnetic field) [40] , the single domain state will remain so after turning off the magnetic field. An interesting question is whether the N =0 state and N =1 skyrmion state need the same critical field to annihilate the skyrmion core (for example, to change the central vortex disk into a single domain state). 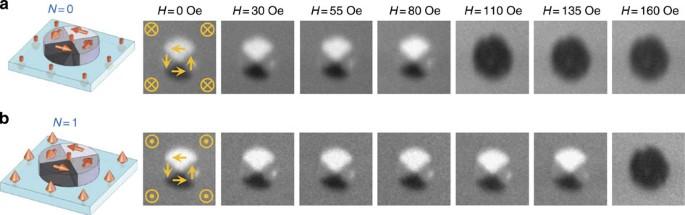Figure 4: The skyrmion PEEM images after applying an in-plane magnetic field pulse. The central vortex is surrounded by out-of-plane Ni spins as indicated by the yellow symbols. (a)N=0 state for parallel alignment between the central vortex core and the surrounding Ni spins, and (b)N=1 skyrmion for antiparallel alignment between the central vortex core and the surrounding Ni spins. The critical field needed to switch the central vortex disk to the single-domain disk (N=0 state) is weaker forN=0 state thanN=1 skyrmion, suggesting a topological effect of in the skyrmion core annihilation process. Figure 4 shows the PEEM images of the central vortex state after application of an in-plane magnetic field pulse of different strengths. The Co spin texture is imaged but, as discussed above, is also representative of the strongly exchange coupled Ni spins. For the N =0 state, the central vortex state remains after the application of an in-plane magnetic field pulse up to ~100 Oe and switches to the single domain state for field greater than ~110 Oe ( Fig. 4a ). In contrast, the N =1 skyrmion central vortex state remains up to a field of ~140 Oe and switches to the single domain state for field greater than ~160 Oe ( Fig. 4b ). As the PEEM images in Fig. 4a,b are taken from the same disk, we attribute the different critical fields in annihilating the skyrmion core to the different topologies of the skyrmion: a lower critical field for N =0 state as opposed to a greater field for N =1 skyrmion. We fabricated and measured 15 samples. Although the critical field varies from sample to sample due to inhomogeneity, we observe the same result that the critical field for N =1 skyrmion is greater than the critical field for N =0 state. Figure 4: The skyrmion PEEM images after applying an in-plane magnetic field pulse. The central vortex is surrounded by out-of-plane Ni spins as indicated by the yellow symbols. ( a ) N =0 state for parallel alignment between the central vortex core and the surrounding Ni spins, and ( b ) N =1 skyrmion for antiparallel alignment between the central vortex core and the surrounding Ni spins. The critical field needed to switch the central vortex disk to the single-domain disk ( N =0 state) is weaker for N =0 state than N =1 skyrmion, suggesting a topological effect of in the skyrmion core annihilation process. Full size image The result can be understood once it is recognized that the spin texture, after the central vortex of a skyrmion becomes a single domain, has a skyrmion number of N =0. Changing the N =0 state into a single-domain disk corresponds to a smooth deformation of the spin texture within the same topological structure, but changing the N =1 skyrmion into a single-domain disk requires a topological change of the spin texture. Therefore, the greater critical field for N =1 skyrmion than N =0 state could be interpreted as the extra field needed to break the topological knot of the N =1 skyrmion. This interpretation is conclusive if the N =0 state and N =1 skyrmion state are energetically degenerate so that the extra field for the N =1 skyrmion has to be associated with a topological barrier. If the N =0 state has a higher energy than the N =1 state (for example, due to the interaction between the skyrmion core and the demagnetization field of the surrounding spins), the greater critical field of the N =1 state might also be explained by different minimum energy evolution traces of the two states. In such a case, there must exist an energy barrier that prevents the transition from the high energy N =0 state to the low energy N =1 skyrmion state before the core annihilation. As this energy barrier originates in the spin interactions and therefore has to be a function of the spin configurations, we could argue that it is the spin texture topology (hidden in the energy barrier) that protects the transition from the N =0 state into the low energy N =1 state. Such a conclusion would require further study to determine other microscopic mechanisms (for example, spinwave emission [41] , external spin-polarized current pulse [25] , [42] , interfacial DM interaction and so on) that also play a role in switching the spin texture topology. Microscopically, as the in-plane magnetic field pushes the skyrmion core to the vortex edge, the N =0 vortex core can enter and disappear in the surrounding out-of-plane spins smoothly, because the core has the same spin direction as the surrounding spins (the initial and final states have the same topology). The N =1 skyrmion core, however, cannot disappear smoothly inside the surrounding spins because of its opposite polarity relative to the environment (the initial and final states have different topologies). That explains why it takes higher critical field to annihilate the N =1 skyrmion core than the N =0 core. From this point of view, our case is similar to the process discussed in refs 22 , 24 and where a spin-polarized current creates/annihilates a single skyrmion [25] , [42] . Finally, we would like to point out that the circulation of the vortex (clockwise or counterclockwise spin curling around the vortex core) is not the topological winding number, which characterizes the spin rotation direction following a counterclockwise contour around the vortex core. The topological winding number is always +1 for vortex state regardless of vortex circulation and is −1 only for an antivortex [27] . We confirmed this assertion by PEEM measurement that N =1 skyrmions of different circulations have the same critical field for skyrmion core annihilation. In conclusion, we realized the artificial magnetic skyrmion proposed in ref. 32 by epitaxially growing a Co disk on top of a perpendicularly magnetized Ni film. We show that the central vortex and the surrounding out-of-plane Ni spins form a magnetic skyrmion whose topology can be tailored between the N =0 and N =1 states by switching the surrounding Ni spin direction relative to the central vortex core polarity. The critical in-plane magnetic field to annihilate the skyrmion core is weaker for N =0 state than for N =1 state, suggesting a topological effect in the skyrmion core annihilation process. Sample fabrication The sample was prepared in an ultrahigh vacuum chamber with a base pressure of 5 × 10 −10 Torr. A Cu(001) substrate was mechanically polished using diamond paste down to 0.25 μm followed by electropolishing. The Cu substrate was treated in the ultrahigh vacuum chamber by cycles of Ar ion sputtering at 2 KeV and annealing at 600 °C. Ni film (30 Ml)was grown epitaxially on top of the Cu(001) substrate at room temperature. The Co was deposited epitaxially at room temperature on top of the 30 Ml Ni film either as a continuous film for MOKE characterization or as disks for skyrmion study, by placing a shadow mask in situ on top of the Ni film. After the Co growth, 2 nm Cu protection layer was grown on top of the sample to prevent contamination. Low-energy electron diffraction) measurement confirms the formation of high-quality single crystalline epitaxial films ( Fig. 1 ). Experimental setup MOKE was used to determine the easy magnetization axis of the continuous Co/Ni(30 Ml)/Cu(001) film. Magnetic hysteresis loops were recorded for magnetic field applied in the out-of-plane and the in-plane directions. A loop with a full remanence shows the easy magnetization character and a loop with zero remanence shows the hard magnetization axis. As the penetration depth of light in metal is ~10 nm, MOKE signal in Fig. 1 represents the hysteresis loop of the whole Co/Ni magnetization. Element-specific XMCD [43] was measured at the Advanced Light Source of Lawrence Berkeley National Lab. on the Co and Ni 2p level at BL6.3.1 for hysteresis loop measurement and at BL11.0.1.1 for PEEM magnetic imaging. Circular polarized X-rays experience different absorption at the 2p L 3,2 edges for magnetization parallel and antiparallel to the X-ray beam, respectively ( Fig. 2b ). Therefore, one can image spin textures with PEEM by taking images of the same area using left- and right-circularly polarized light at an appropriate energy and dividing one image by the other. The resulting PEEM XMCD image exhibits intensity contrast for different spin orientations within the sample plane (bright, grey and dark for spins parallel, perpendicular and antiparallel, respectively, to the X-ray beam). The lateral magnetic spatial resolution of PEEM is ~50–100 nm so that PEEM measurement cannot resolve the out-of-plane magnetic vortex core. Micromagnetic simulation Micromagnetic simulation was carried out using the Object Oriented MicroMagnetic Framework code [44] based on the Landau–Lifshitz–Gilbert equation. The model contains a Co disk on top of a continuous Ni film with the same parameters as our experimental system: saturation magnetization M S,Co =1.4 × 10 6 A m −1 ; exchange stiffness A Co =3 × 10 −11 J m −1 ; Co thickness t Co =30 nm; in-plane fourfold magnetic anisotropy [45] K Co =8 × 10 4 J m −3 for Co and M S,Ni =4.9 × 10 5 A m −1 ; A Ni =1.2 × 10 −11 J m −1 ; t Ni =5 nm for Ni layer. The cell size is 2 × 2 × 2.5 nm in our simulation. The Ni film perpendicular anisotropy, K ⊥ =3.5 × 10 5 J m −3 is obtained from the equation of , where H S is the saturating field of Ni in-plane hysteresis loop ( Fig.2 ). A Co/Ni interfacial coupling of A Co/Ni =2 × 10 −11 J m −1 is adapted, but the result is insensitive to A Co/Ni value at lease in the range of A Ni < A Co/Ni < A Co . 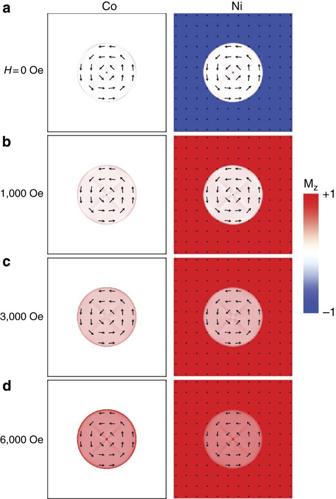Figure 5: Simulation result of the Co and Ni domains within different out-of-plane magnetic fields. (a)H=0 Oe; (b)H=1000 Oe; (c)H=3000 Oe; (d)H=6000 Oe. The surrounding out-of-plane Ni spins switch from −zto +zdirections aboveH=800 Oe, but the central vortex core switches its polarity from −zto +zdirections atH=6,000Oe. This allows the switching of the skyrmion topology betweenN=0 andN=1 states by switching the surrounding Ni spin direction using an 800-Oe out-of-plane magnetic field without switching the central vortex core polarity. Figure 5a shows the simulation result after removing 2.0 T magnetic field in the − z direction. The Co disk forms the expected vortex state with its core polarity in the − z direction. The Ni spins form a skyrmion with the central vortex following the vortex structure of the Co disk and the Ni spins outside the disk region in the − z direction (plus a domain wall between the central vortex and the outside spins). Subsequent simulations are performed when H =1,000 Oe static magnetic field is applied in the + z direction. It can be clearly seen that the outside out-of-plane Ni spins are switched from − z to + z directions, but the central vortex core remains in the − z direction ( Fig. 5 ). After this state, we performed two simulations. One simulation is to release the H =1,000 Oe field to get the remanent state ( N =1 skyrmion shown in Fig. 3c ). The other is the simulation by increasing the magnetic field in the + z direction. We find that the central vortex core remains in the −z direction (blue dot at the core position, see Fig. 5 ) until H =6,000 Oe where the central vortex core switches to the + z direction (red dot at the core position, see Fig. 5 ). Figure 5: Simulation result of the Co and Ni domains within different out-of-plane magnetic fields. ( a ) H =0 Oe; ( b ) H =1000 Oe; ( c ) H =3000 Oe; ( d ) H =6000 Oe. The surrounding out-of-plane Ni spins switch from − z to + z directions above H =800 Oe, but the central vortex core switches its polarity from − z to + z directions at H =6,000Oe. This allows the switching of the skyrmion topology between N =0 and N =1 states by switching the surrounding Ni spin direction using an 800-Oe out-of-plane magnetic field without switching the central vortex core polarity. Full size image How to cite this article: Li, J. et al. Tailoring the topology of an artificial magnetic skyrmion. Nat. Commun. 5:4704 doi: 10.1038/ncomms5704 (2014).